PBX3 is targeted by multiple miRNAs and is essential for liver tumour-initiating cells Tumour-initiating cells (TICs) are advocated to constitute the sustaining force to maintain and renew fully established malignancy; however, the molecular mechanisms responsible for these properties are elusive. We previously demonstrated that voltage-gated calcium channel α2δ1 subunit marks hepatocellular carcinoma (HCC) TICs. Here we confirm directly that α2δ1 is a HCC TIC surface marker, and identify let-7c, miR-200b, miR-222 and miR-424 as suppressors of α2δ1 + HCC TICs. Interestingly, all the four miRNAs synergistically target PBX3 , which is sufficient and necessary for the acquisition and maintenance of TIC properties. Moreover, PBX3 drives an essential transcriptional programme, activating the expression of genes critical for HCC TIC stemness including CACNA2D1 , EpCAM, SOX2 and NOTCH3 . In addition, the expression of CACNA2D1 and PBX3 mRNA is predictive of poor prognosis for HCC patients. Collectively, our study identifies an essential signalling pathway that controls the switch of HCC TIC phenotypes. As a highly tumorigenic and drug-resistant subpopulation, tumour-initiating cells (TICs) or cancer stem cells (CSCs) own many stem cell-like properties such as self-renewal and differentiation [1] , [2] , [3] . TICs are able to generate the heterogeneous lineages of cancer cells that comprise the tumour, and hence have been advocated to constitute the sustaining force to maintain and renew fully established malignancy. These properties of TICs have therefore led to the proposal that TICs are responsible for tumour occurrence, metastasis and recurrence, and TIC-targeted therapeutic approaches may provide promising strategies to improve clinical cancer therapy [4] . Although exactly how TICs emerge remains elusive, accumulating evidence demonstrates that TICs may be the oncogenic derivatives of normal-tissue stem or progenitor cells, or arise from acquisition of stem cell properties by more differentiated cells as a result of transformation-associated genetic or epigenetic reprogramming [5] , [6] , [7] , [8] , [9] , [10] . Furthermore, recent studies indicate that CSC phenotypes can reversibly turn on and off spontaneously or with the variation of their microenvironment niches [11] , [12] , [13] , [14] . Uncovering the molecular pathways involved in the control of TIC properties is critical for the understanding of TIC biology as well as for the development of novel therapies [3] . However, functional identification of such molecules at genome-wide scale is usually hindered by the limited availability and unstable properties of TICs. MicroRNAs (miRNA), a large family of short noncoding RNAs that negatively regulate mRNA stability or translation through imperfect base pairing with the 3′-untranslated regions (UTRs) of target genes, have been functionally linked to stem cells [15] , [16] , [17] , [18] and TICs or CSCs [19] . In fact, aberrant expression of miRNAs such as let-7, miR-34a, miR-181a, miRNA-130b in TICs has been found in a variety of tumour types. These aberrantly expressed miRNAs play essential roles in the regulation of TIC properties as either TIC suppressors or promoters [20] , [21] , [22] , [23] , [24] . Moreover, a series of critical signalling pathways involved in the regulation of TIC properties have been uncovered with the identification of the targets of these miRNAs [19] , [25] , [26] , [27] , [28] . Importantly, miRNAs are also demonstrated to be promising biomarkers and amenable therapeutic targets [5] , [19] , [24] . On the basis of a pair of hepatocellular carcinoma (HCC) cell lines Hep-11 and Hep-12, which represent non-tumorigenic and TIC-enriched cell populations, respectively [29] , we identified a subpopulation of TICs expressing the isoform 5 of the voltage-gated calcium channel α2δ1 subunit (encoded by the gene CACNA2D1 ), which is vital for the activation of calcium signalling that controls the HCC TIC properties using an antibody, Mab1B50-1, generated against Hep-12 cells [30] , [31] . Here we first validate directly that α2δ1 is indeed a surface marker for HCC TICs using a known α2δ1 antibody and identify its prognostic role in HCC. Subsequently, we identify 4 α2δ1 + TIC suppressor miRNAs (let-7c, miR-200b, miR-222 and miR-424) that synergistically target PBX3, which is essential for α2δ1 + HCC TIC properties through genome-wide miRNA profiling of Hep-11 and Hep-12 cells, followed by soft-agar formation functional screening. Our studies indicate that downregulation of the four miRNAs is responsible for the acquisition and subsequent maintenance of α2δ1 + TIC phenotypes via common target PBX3, which serves as a transcriptional switch between TIC and non-TIC programming. Confirmation of α2δ1 as a HCC TIC marker To directly confirm that α2δ1 is a surface marker that marks HCC TICs, we purified both α2δ1 + and α2δ1 − cells using a known α2δ1 antibody using fluorescence-activated cell sorting (FACS) from HCC cell lines, including Huh7, HepG2, SMMC7721, as well as primary HCC tissues to assay their self-renewal and tumorigenic properties. As shown in Fig. 1a,b , purified α2δ1 + cells formed spheres in serum-free medium at significantly higher rates than their negative counterparts. Furthermore, single cells obtained from these α2δ1 + -dissociated spheres could be clonally expanded and serially propagated, demonstrating that these α2δ1 + cells possess in vitro self-renewal capability. 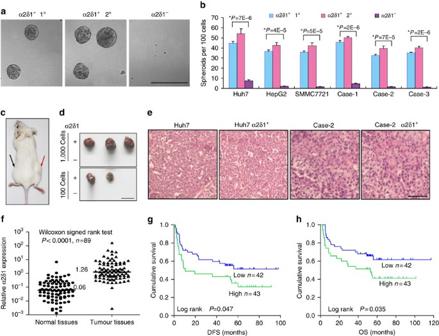Figure 1: The tumour-initiating properties of α2δ1+HCC cells. (a) Phase contrast micrographs demonstrate that FACS-sorted α2δ1+Huh7 cells are able to form more primary (1°) and serially passaged (2°) spheroids as compared with α2δ1−counterparts. Scale bar, 250 μm. (b) Histograms show the primary (1°) and serially passaged (2°) spheroid formation efficiency of the α2δ1+cells as compared with α2δ1−cells sorted from indicated sources. Bars are the mean±s.d. of three independent experiments (n=6). * Student’st-test. (c) Representative photograph showing tumour formation in NOD/SCID mice was restricted to the α2δ1+cell population (red arrow). No tumour growth was usually observed on injection of α2δ1−cells (black arrow) on the opposite flanks of the same animals. (d) Representative images showing the dissected tumours formed by sorted α2δ1+Huh7 cells. A total of three mice per group were transplanted. Scale bar, 2 cm. (e) The histology of tumours formed by α2δ1+cells purified from a primary HCC tissue (Case-2) and Huh7 cell line was compared with that of original patient tumour and parent Huh7 tumour, respectively, by HE staining. Scale bar, 100 μm. (f) qRT–PCR analysis of α2δ1 mRNA levels in HCC tissues and paired normal tissues adjacent to tumours. Horizon lines indicate the median values of each group. (g,h) Kaplan–Meier curves for the disease-free survival (DFS) and overall survival (OS) of 85 HCC patients were compared between groups with high and low levels of α2δ1 mRNA in HCC tissues, which were divided according to the cutoff of 1.26, the median value of α2δ1 relative toGAPDHmRNA. Figure 1: The tumour-initiating properties of α2δ1 + HCC cells. ( a ) Phase contrast micrographs demonstrate that FACS-sorted α2δ1 + Huh7 cells are able to form more primary (1°) and serially passaged (2°) spheroids as compared with α2δ1 − counterparts. Scale bar, 250 μm. ( b ) Histograms show the primary (1°) and serially passaged (2°) spheroid formation efficiency of the α2δ1 + cells as compared with α2δ1 − cells sorted from indicated sources. Bars are the mean±s.d. of three independent experiments ( n =6). * Student’s t -test. ( c ) Representative photograph showing tumour formation in NOD/SCID mice was restricted to the α2δ1 + cell population (red arrow). No tumour growth was usually observed on injection of α2δ1 − cells (black arrow) on the opposite flanks of the same animals. ( d ) Representative images showing the dissected tumours formed by sorted α2δ1 + Huh7 cells. A total of three mice per group were transplanted. Scale bar, 2 cm. ( e ) The histology of tumours formed by α2δ1 + cells purified from a primary HCC tissue (Case-2) and Huh7 cell line was compared with that of original patient tumour and parent Huh7 tumour, respectively, by HE staining. Scale bar, 100 μm. ( f ) qRT–PCR analysis of α2δ1 mRNA levels in HCC tissues and paired normal tissues adjacent to tumours. Horizon lines indicate the median values of each group. ( g , h ) Kaplan–Meier curves for the disease-free survival (DFS) and overall survival (OS) of 85 HCC patients were compared between groups with high and low levels of α2δ1 mRNA in HCC tissues, which were divided according to the cutoff of 1.26, the median value of α2δ1 relative to GAPDH mRNA. Full size image Next, we transplanted serially diluted α2δ1 + and α2δ1 − cells subcutaneously (s.c.) into nonobese diabetes/severe combined immunodeficient (NOD/SCID) mice to evaluate their tumorigenic potential. As few as 100 purified α2δ1 + cells from HCC cell lines and primary tumours were able to initiate tumour formation in almost all of the transplanted mice in 8 weeks following transplantation, whereas the α2δ1 − cells were not observed for any nodules formed within 12 weeks ( Fig. 1c,d ; Table 1 ; Supplementary Fig. 1 ). In addition, when α2δ1 + and α2δ − cells sorted from these primary tumour xenografts were retransplanted into secondary mouse recipients, only α2δ1 + cells successfully resulted in tumour formation, indicating that tumorigenic α2δ1 + cells have the in vivo self-renewal potential ( Table 1 ; Supplementary Fig. 1 ). Histological analysis with the tumours formed by α2δ1 + cells by haematoxylin and eosine (HE) staining showed that the tumour morphologies are indistinguishable from their parent cells ( Fig. 1e ). Table 1 Engraftment rates of α2δ1 + and α2δ1 − subpopulations in NOD/SCID mice. Full size table These data, along with our previous results with Mab1B50-1 (ref. 30 ), demonstrate clearly that a TIC population with stem cell-like properties in HCC could be defined by a surface α2δ1 phenotype. Clinical significance of α2δ1 expression in HCC Since TICs are usually rare in tumour tissues, it is hard to quantify the immunohistochemical staining results. We therefore performed quantitative reverse transcription–polymerase chain reaction (qRT–PCR) analysis in 89 paired HCC and adjacent normal tissues to test the clinical significance of α2δ1. The α2δ1 mRNA level in cancer tissues was remarkably higher than that of matched normal tissues ( Fig. 1f ). Further analysis of α2δ1 mRNA expression in cancer tissues from 85 HCC patients with detailed follow-up information showed that high level of α2δ1 mRNA was positively correlated not only with tumour size, but also with rapid recurrence and short overall survival post surgery ( Supplementary Table 1 ). Kaplan–Meier survival curves showed that the patients with high level of α2δ1 mRNA displayed both shorter tumour-free survival ( Fig. 1g ) and overall survival periods ( Fig. 1h ). 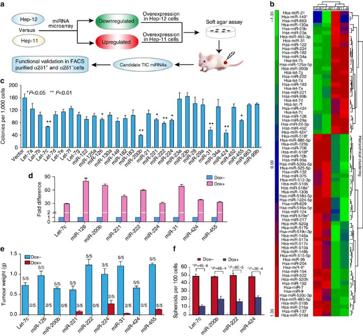Figure 2: Identification of candidate miRNAs that control α2δ1+HCC TICs. (a) Schematic overview of the strategy for identification of α2δ1+HCC TIC miRNAs based on the Hep-11 and Hep-12 cell lines. (b) Heat map of miRNA expression showing the miRNAs deregulated in the TIC-enriched Hep-12 cells versus the non-tumorigenic Hep-11 cells (P<0.01). Clustering was performed with average linkage and uncentred correlation using the Partek Genomics Suite (Partek SG Pte Ltd, Singapore). (c) The effect of indicated miRNAs on the colony formation efficiency of Hep-12 cells in soft agar. Pools of Hep-12 cells stably transfected with each indicated pri-mRNA were plated into 0.3% agar at 1,000 cells per well (n=6). Error bars represent s.d. **Student’st-test. (d) qRT–PCR results demonstrate that the indicated miRNAs are induced significantly at 48 h after 2 μg ml−1DOX was added into the culture medium of Hep-12 cells, which were stably infected with tet-on pri-miRNA expression lentiviruses. Error bars represent s.d. (e). Tumour formation by Hep-12 cells stably infected with inducible pri-miRNA expression lentiviruses were assayed after transplanting 104cells in Matrigel subcutaneously. To induce the miRNA expression, mice in the DOX(+) group were fed with water containing 2 mg ml−1DOX. The numbers above each bar indicate the tumour-formation rates that are expressed as tumours formed/sites transplanted. (f) The spheroid formation efficiency of Hep-12 cells after the expression of indicated miRNAs was induced with 2 μg ml−1DOX (n=6). Data are means±s.d. of three independent experiments. *Student’st-test. Cox regression analysis also identified that high level of α2δ1 mRNA is an independent risk factor of poor survival for HCC patients (relative risk=2.66, P =0.005, Supplementary Table 2 ), suggesting that the α2δ1 mRNA level in HCC may serve as a prognostic factor. Identification of miRNAs that suppress Hep-12 cell stemness To find miRNAs that regulate the stemness of HCC TICs, we took advantage of the TIC-enriched Hep-12 and the non-tumorigenic Hep-11 cell lines by genome-wide profiling of miRNA expression with miRNA microarray analysis, followed by functional screening with soft-agar assay ( Fig. 2a ). Figure 2: Identification of candidate miRNAs that control α2δ1 + HCC TICs. ( a ) Schematic overview of the strategy for identification of α2δ1 + HCC TIC miRNAs based on the Hep-11 and Hep-12 cell lines. ( b ) Heat map of miRNA expression showing the miRNAs deregulated in the TIC-enriched Hep-12 cells versus the non-tumorigenic Hep-11 cells ( P <0.01). Clustering was performed with average linkage and uncentred correlation using the Partek Genomics Suite (Partek SG Pte Ltd, Singapore). ( c ) The effect of indicated miRNAs on the colony formation efficiency of Hep-12 cells in soft agar. Pools of Hep-12 cells stably transfected with each indicated pri-mRNA were plated into 0.3% agar at 1,000 cells per well ( n =6). Error bars represent s.d. **Student’s t -test. ( d ) qRT–PCR results demonstrate that the indicated miRNAs are induced significantly at 48 h after 2 μg ml −1 DOX was added into the culture medium of Hep-12 cells, which were stably infected with tet-on pri-miRNA expression lentiviruses. Error bars represent s.d. ( e ). Tumour formation by Hep-12 cells stably infected with inducible pri-miRNA expression lentiviruses were assayed after transplanting 10 4 cells in Matrigel subcutaneously. To induce the miRNA expression, mice in the DOX(+) group were fed with water containing 2 mg ml −1 DOX. The numbers above each bar indicate the tumour-formation rates that are expressed as tumours formed/sites transplanted. ( f ) The spheroid formation efficiency of Hep-12 cells after the expression of indicated miRNAs was induced with 2 μg ml −1 DOX ( n =6). Data are means±s.d. of three independent experiments. *Student’s t -test. Full size image Comparing with Hep-11 cells, 31 mature miRNAs including those that have been reported to have a tumour-suppressor role in other types of TICs such as let-7 family members, miR-200b and miR-34a, were found to be downregulated, and 46 mature miRNAs including miR-130b, which acted as an oncomir in CD133 + HCC TICs [21] , were upregulated significantly in Hep-12 cells ( Fig. 2b ). Each expression construct of those downregulated miRNAs was then transfected into Hep-12 cells, and the G418-resistant cell pools were assayed for their abilities to grow in soft agar. A total of nine miRNAs including let-7c, mir-126, mir-200b, mir-221, mir-222, mir-224, mir-31, mir-424 and mir-455 were able to inhibit the colony formation of Hep-12 cells significantly compared with the vector alone control ( P <0.05, Fig. 2c ). Tetracycline-inducible Hep-12 cells expressing each of the above nine miRNAs were further established by employing the TET-on lentiviral system ( Fig. 2d ), and 10 4 cells per mouse were injected s.c. into NOD/SCID mice to evaluate the change of tumorigenic property after doxocycline (DOX) was administrated in drinking water. Interestingly, induced expression of these nine miRNAs could remarkably retard in vivo tumour growth of Hep-12 cells, while let-7c, miR-200b, miR-222 and miR-424 resulted in a complete inhibition of tumour formation ( Fig. 2e ). The four most effective miRNAs, let-7c, miR-200b, miR-222 and miR-424, were further tested for their effects on the self-renewal ability of Hep-12 cells by spheroid formation assay. The spheroid formation efficiency decreased significantly when the expression of the four miRNAs was induced individually by DOX ( P ≤0.001, Fig. 2f ). Therefore, we have identified four miRNAs, let-7c, miR-200b, miR-222 and miR-424, which are downregulated in Hep-12 cells and are able to suppress the self-renewal and tumorigenic properties of Hep-12 cells. The suppression roles of the four miRNAs on HCC TICs To validate that these four miRNAs are indeed involved in the regulation of α2δ1 + HCC TICs in general, we first detected their expression in FACS-purified α2δ1 + and α2δ1 − subsets using qRT–PCR. As expected, the four miRNAs were found to be remarkably downregulated in α2δ1 + subsets from a variety of HCC cell lines and primary tissues comparing with their α2δ1 − counterparts ( Fig. 3a ). The downregulation of the four miRNAs in α2δ1 + TICs was further confirmed by miRNA fluorescence in situ hybridization ( Supplementary Fig. 2 ). 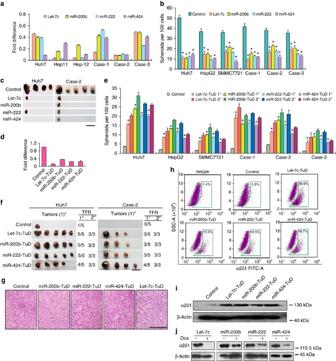Figure 3: The effects of let-7c, miR-200b, miR-222 and miR-424 on the self-renewal and tumorigenicity of HCC TICs. (a) The expression of indicated miRNAs in α2δ1+and α2δ−cells purified from indicated sources were detected using qRT–PCR. The data presented as fold difference of α2δ1+cells over α2δ−counterparts that was defined as 1 (omitted in the histogram). Error bars indicate s.d. (b,c) FACS-sorted α2δ1+fractions were incubated with indicated lentiviruses for 2 h and were plated in 96-well plates at 100 cells per well (n=6) to assay their spheroid formation efficiency (b), or were transplanted into NOD/SCID mice (n=5) at 1,000 cells per site to test their tumorigenicity (c). Scale bar, 2 cm. Data in (b) are means±s.d. of three independent experiments. *Student’st-test,P<0.01 versus respective controls. (d) The fold difference (2−ΔΔCt) of indicated miRNAs in Huh7 α2δ1−cells following TuD RNA interference of the indicated miRNAs over the control (infected with empty virus), which was set up as 1. Error bars indicate s.d. of three experiments. (e,f) FACS-sorted α2δ1−cells were infected with lentiviruses harbouring TuD RNA expression constructs against indicated miRNAs and were subsequently plated into 96-well plates to assay their primary spheroid formation efficiency (1°) and subsequent expansion ability (2°,e;n=6), or serially transplanted s.c. into NOD/SCID mice at 1,000 cells per site (f;n=5). Scale bar, 2 cm. TFR, tumour-formation rate that is expressed as tumours formed/sites transplanted. Data in (e) are means±s.d. of three independent experiments. *Student’st-test,P<0.01 versus respective controls. (g) HE staining demonstrating the histology of the tumours formed inf. Scale bar, 150 μm. (h) The frequencies of α2δ1+cells were measured by flow cytometry in Huh7 cells after indicated miRNAs were knocked down by infection with Tud RNA lentiviruses. The data are representative of three experiments. (i,j) Western blot analysis of α2δ1 expression in Huh7 cells after indicated miRNAs were knocked down (i) and in Hep-12 cells after induced expression of indicated miRNAs (j). Figure 3: The effects of let-7c, miR-200b, miR-222 and miR-424 on the self-renewal and tumorigenicity of HCC TICs. ( a ) The expression of indicated miRNAs in α2δ1 + and α2δ − cells purified from indicated sources were detected using qRT–PCR. The data presented as fold difference of α2δ1 + cells over α2δ − counterparts that was defined as 1 (omitted in the histogram). Error bars indicate s.d. ( b , c ) FACS-sorted α2δ1 + fractions were incubated with indicated lentiviruses for 2 h and were plated in 96-well plates at 100 cells per well ( n =6) to assay their spheroid formation efficiency ( b ), or were transplanted into NOD/SCID mice ( n =5) at 1,000 cells per site to test their tumorigenicity ( c ). Scale bar, 2 cm. Data in ( b ) are means±s.d. of three independent experiments. *Student’s t -test, P <0.01 versus respective controls. ( d ) The fold difference (2 −ΔΔ C t ) of indicated miRNAs in Huh7 α2δ1 − cells following TuD RNA interference of the indicated miRNAs over the control (infected with empty virus), which was set up as 1. Error bars indicate s.d. of three experiments. ( e , f ) FACS-sorted α2δ1 − cells were infected with lentiviruses harbouring TuD RNA expression constructs against indicated miRNAs and were subsequently plated into 96-well plates to assay their primary spheroid formation efficiency (1°) and subsequent expansion ability (2°, e ; n =6), or serially transplanted s.c. into NOD/SCID mice at 1,000 cells per site ( f ; n =5). Scale bar, 2 cm. TFR, tumour-formation rate that is expressed as tumours formed/sites transplanted. Data in ( e ) are means±s.d. of three independent experiments. *Student’s t -test, P <0.01 versus respective controls. ( g ) HE staining demonstrating the histology of the tumours formed in f . Scale bar, 150 μm. ( h ) The frequencies of α2δ1 + cells were measured by flow cytometry in Huh7 cells after indicated miRNAs were knocked down by infection with Tud RNA lentiviruses. The data are representative of three experiments. ( i , j ) Western blot analysis of α2δ1 expression in Huh7 cells after indicated miRNAs were knocked down ( i ) and in Hep-12 cells after induced expression of indicated miRNAs ( j ). Full size image We then overexpressed the four miRNAs individually in FACS-purified α2δ1 + TICs from HCC cell lines and primary tissues to test their effects on the self-renewal capability. Forced expression any of the four miRNAs resulted in remarkable inhibition of spheroid formation of α2δ1 + cells, indicating that these miRNAs could suppress the in vitro self-renewal ability of α2δ1 + HCC TICs ( Fig. 3b ). Next, 1,000 sorted α2δ1 + cells from Huh7 cell line and a patient biopsy, which were incubated with lentiviruses harbouring each of the four miRNAs, were transplanted s.c. into NOD/SCID mice to test their tumorigenicity. Comparing with the control lentivirus-infected cells, the tumorigenicity of α2δ1 + TICs was significantly suppressed with any of the four miRNAs overexpressed ( Fig. 3c ). Hence, let-7c, miR-200b, miR-222 and miR-424 could indeed suppress the self-renewal and tumorigenic properties of α2δ1 + TICs. The knockdown effects of the four miRNAs We furthered our study to test whether the downregulation of the four miRNAs individually is sufficient to convert α2δ1 − cells into TIC-like cells by knockdown of the four miRNAs individually using the tough decoy (TuD) RNA method [32] . The expression of let-7c, miR-200b, miR-222 and miR-424 was inhibited ∼ 89.3%, 64.3%, 76.6% and 75.0%, respectively, in α2δ1 − cells purified from Huh7 cells by TuD RNAs against each miRNA compared with control ( Fig. 3d ). Next, we performed spheroid formation assay to measure whether the α2δ1 − cells could acquire in vitro self-renewal ability following these miRNAs’ knockdown. The spheroid formation efficiency of α2δ1 − cells was remarkably promoted following knockdown of the four miRNAs individually. Furthermore, single cells obtained from these dissociated spheres could be clonally expanded in subsequent serial propagations with increased efficiency, demonstrating that these α2δ1 − cells acquired in vitro self-renewal capability after individual knockdown of the four miRNAs. Similar results were obtained when the four miRNAs were interfered in α2δ1 − cells purified from more HCC cell lines and primary tissues ( Fig. 3e ). We then transplanted 10 3 α2δ1 − cells purified from the Huh7 cell line and a primary HCC tissue into NOD/SCID mice to evaluate their tumorigenicity following individual knockdown of the four miRNAs. Newly acquired or enhanced tumorigenicity was observed for α2δ1 − cells after knockdown any of these four miRNAs. Furthermore, these primary xenografted tumours could also self-renew, as demonstrated by their ability to form new tumours when serially transplanted in secondary mouse recipients ( Fig. 3f ). HE staining confirmed that the tumours formed were of HCC histology ( Fig. 3g ). Finally, we checked the expression of the TIC surface marker α2δ1 after knockdown of the four miRNAs. As shown in Fig. 3h , clear subpopulations of α2δ1 + cells emerged on individual knockdown of the four miRNAs in α2δ1 − Huh7 cells. Furthermore, western blot analyses demonstrated that the expression of α2δ1 was also upregulated after knockdown of each of the four miRNAs ( Fig. 3i ). On the contrary, the expression of α2δ1 decreased significantly in Hep-12 cells on the switch of let-7c, miR-200b, miR-222 and miR-424 expression ( Fig. 3j ). Therefore, knockdown the four miRNAs individually was sufficient to convert α2δ1 − cells into TICs with stem cell-like properties. PBX3 is a bonafide common target of the four miRNAs Given that all the four miRNAs can suppress the properties of α2δ1 + HCC TICs, we hypothesized that the common genes directly targeted by them may play central roles in the determination of HCC TIC properties. Indeed, seven genes, including ADRBK2 , HIPK2 , PBX3 , PLEKHA6 , PRKAB2 , RIMS3 and TAF9B , were found to be potential common targets of the four miRNAs ( Fig. 4a ) by merging the list of upregulated genes in the α2δ1 + TICs obtained by Affymetrix microarray mRNA hybridization (our unpublished data) with predicted target genes of each of the four miRNAs using the miRWalk algorithm [33] . 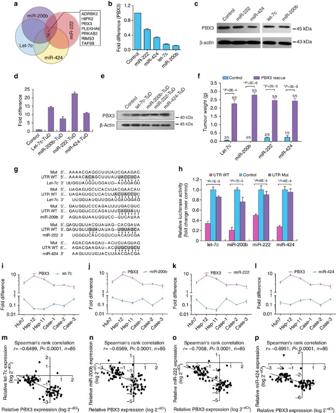Figure 4:PBX3is a common target of let-7c, miR-200b, miR-222 and miR-424. (a) Venn diagram shows candidate mRNAs that were predicted to be directly targeted by all the four miRNAs byin silicoanalysis of upregulated genes in the α2δ1+HCC TICs with predicted target genes of each of the four miRNAs using the miRWalk algorithm. (b,c) qRT–PCR and western blot assays were carried out to detect the expression of endogenousPBX3at both mRNA (b) and protein (c) levels, respectively, in Hep-12 cells infected with lentiviruses harboring indicated miRNAs. (d,e) The expression of endogenousPBX3at both mRNA (d) and protein (e) levels in FACS-sorted α2δ1−Huh7 cells after indicated miRNAs were knocked down by TuD RNAs. (f) The effects ofPBX3on tumour formation of Hep-12 cells expressing indicated miRNAs. The numbers above each bar indicate the tumour-formation rates that are expressed as tumours formed/sites transplanted. The bars are means±s.d. of tumour weights. *Student’st-test. (g) Sequence alignment of the seed sequence of indicated miRNAs with portions of thePBX33′-UTR (UTR WT) as predicted using the TargetScan software. The sequences designed as ‘Mut’ are mutated sequences in the matched seed sites that were used for creating firefly luciferase reporter constructs. (h) Dual-luciferase reporter assay in Hep-12 cells transiently co-transfected with the indicated constructs. Data are the average±s.d. of three independent experiments. *Student’st-test. (i–l) The inverse correlation of indicated miRNAs againstPBX3mRNA expression was determined across purified α2δ1+and α2δ1−subsets from indicated sources. Data represented fold difference of α2δ1+cells over their negative counterparts in the same categories. Error bars indicate s.d. of three independent experiments. (m–p) The relationship between the expression of indicated miRNAs andPBX3mRNA in clinical HCC tissues. Figure 4: PBX3 is a common target of let-7c, miR-200b, miR-222 and miR-424. ( a ) Venn diagram shows candidate mRNAs that were predicted to be directly targeted by all the four miRNAs by in silico analysis of upregulated genes in the α2δ1 + HCC TICs with predicted target genes of each of the four miRNAs using the miRWalk algorithm. ( b , c ) qRT–PCR and western blot assays were carried out to detect the expression of endogenous PBX3 at both mRNA ( b ) and protein ( c ) levels, respectively, in Hep-12 cells infected with lentiviruses harboring indicated miRNAs. ( d , e ) The expression of endogenous PBX3 at both mRNA ( d ) and protein ( e ) levels in FACS-sorted α2δ1 − Huh7 cells after indicated miRNAs were knocked down by TuD RNAs. ( f ) The effects of PBX3 on tumour formation of Hep-12 cells expressing indicated miRNAs. The numbers above each bar indicate the tumour-formation rates that are expressed as tumours formed/sites transplanted. The bars are means±s.d. of tumour weights. *Student’s t -test. ( g ) Sequence alignment of the seed sequence of indicated miRNAs with portions of the PBX3 3′-UTR (UTR WT) as predicted using the TargetScan software. The sequences designed as ‘Mut’ are mutated sequences in the matched seed sites that were used for creating firefly luciferase reporter constructs. ( h ) Dual-luciferase reporter assay in Hep-12 cells transiently co-transfected with the indicated constructs. Data are the average±s.d. of three independent experiments. *Student’s t -test. ( i – l ) The inverse correlation of indicated miRNAs against PBX3 mRNA expression was determined across purified α2δ1 + and α2δ1 − subsets from indicated sources. Data represented fold difference of α2δ1 + cells over their negative counterparts in the same categories. Error bars indicate s.d. of three independent experiments. ( m – p ) The relationship between the expression of indicated miRNAs and PBX3 mRNA in clinical HCC tissues. Full size image PBX3 belongs to the highly conserved PBX (Pre-B-cell leukaemia homeobox) group of proteins, which in turn belongs to the PBC family of TALE (three-amino-acid loop extension) superclass of homeodomain proteins. It appears to be the most critical member of PBX family contributing to leukaemogenesis by serving as a cofactor of other homeodomain proteins such as HOX and MEIS [34] , [35] to control gene expression, and has been identified as a direct target of let-7c, miR-181a/miR-181b, to function in colorectal cancer metastasis and leukaemogenesis, respectively [36] , [37] . Hence, PBX3 was chosen to validate further whether it was directly targeted by the four miRNAs to regulate α2δ1 + HCC TICs. We first tested whether the expression of PBX3 was negatively regulated by the four miRNAs. Compared with respective controls, the expression of PBX3 decreased remarkably at both mRNA and protein levels when the four miRNAs were overexpressed individually in Hep-12 cells by lentivirus infection ( Fig. 4b,c ). Conversely, the expression of PBX3 increased significantly after each of the four miRNAs was interfered in α2δ1 − Huh7 cells at both mRNA and protein levels ( Fig. 4d,e ). Rescue experiments were then performed to validate whether PBX3 could functionally overcome the suppression effects of the four miRNAs on HCC TICs. Ectopic expression of PBX3 in Hep-12 cells individually overexpressed the four miRNAs resulted in tumorigenicity recovered when 10 3 cells per site were transplanted into NOD/SCID mice ( Fig. 4f ), confirming that downregulation of PBX3 is necessary for the suppression roles of the four miRNAs. Luciferase reporter assay was further carried out by employing a luciferase reporter vector containing the 3′-UTR of PBX3 flanking all the putative binding sites of the four miRNAs. Mutations in the putative binding sites were created as controls ( Fig. 4g ). When each of the four miRNAs was co-transfected with the reporter vector, the luciferase activities of the wild-type (WT) 3′-UTRs of PBX3 were inhibited significantly compared with the respective mutant constructs ( Fig. 4h ). Finally, the correlation between the expression of the four miRNAs and PBX3 mRNA was analysed in purified α2δ1 + and α2δ1 − fractions, as well as in clinical HCC samples. As expected, PBX3 mRNA levels were negatively correlated with those of let-7c, miR-200b, miR-222 and miR-424 in purified α2δ1 + and α2δ1 − fractions across HCC cell lines and primary tissues ( Fig. 4i–l ), as well as in unsorted HCC samples ( Fig. 4m–p ). These data indicate that the four miRNAs could suppress individually the properties of α2δ1 + HCC TICs by directly targeting PBX3 . PBX3 determines the α2δ1 + HCC TIC phenotypes The above results prompted us to pursue further whether PBX3 plays some roles in the acquisition and/or maintenance of HCC TIC properties. We first compared the expression of PBX3 between Hep-12 and Hep-11 cell lines, and between the α2δ1 + and α2δ1 − fractions sorted from HCC cell lines and primary HCC tissues. Indeed, the expression of PBX3 was higher in Hep-12 cells than in Hep-11 cells, and was preferentially expressed in α2δ1 + HCC TICs as compared with their negative counterparts at both mRNA and protein levels ( Fig. 5a–d ). 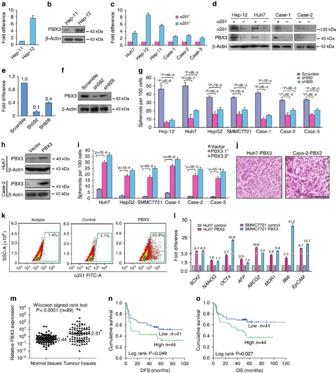Figure 5:PBX3is a critical determinant of α2δ1+HCC TICs. (a,b) The expression ofPBX3in Hep-11 and Hep-12 cells was detected at both mRNA and protein levels using qRT–PCR (a) and western blot (b), respectively. (c,d) The expression ofPBX3was compared between α2δ1+and α2δ1−fractions from indicated sources at both mRNA (c) and protein levels (d). (e,f) qRT–PCR (e) and western blot (f) results showing the knockdown effects ofPBX3shRNAs on the expression ofPBX3in Hep-12 cells at both mRNA and protein levels. β-actin serves as an internal control. (g) Sorted α2δ1+cells from indicated sources were infected with lentiviruses harbouringPBX3shRNAs, followed by plating 100 cells per well into 96-well plates to assay their sphere formation potential (n=6). Data are the average±s.d. of three independent experiments. *Student’st-test. (h) α2δ1−cells from indicated sources were infected withPBX3lentivirus and assayed for PBX3 by western blot. (i) FACS-sorted α2δ1−cells from indicated sources were infected withPBX3lentivirus and assayed for their sphere formation ability (n=6). Data are the average±s.d. of three independent experiments. *Student’st-test. (j) HE staining showing the histology of the tumours formed by α2δ1−cells from indicated sources afterPBX3lentivirus infection. Scale bar, 100 μm. (k) The percentage of α2δ1-positive cells were measured using flow cytometry inPBX3-lentivirus-infected Huh7 α2δ1−cells compared. with vector alone control. The data are representative of three experiments. (l) The expression of stem cell-related genes in α2δ1−cells overexpressing PBX3 was compared with vector alone controls using qRT–PCR. (m) The expression ofPBX3mRNA in HCC tissues was compared with adjacent normal tissues using qRT–PCR. *The numbers next to the horizontal lines are the median values (2−ΔCt) for each group. (n,o) Kaplan–Meier curves for the DFS and OS of patients were compared between groups with high and low levels ofPBX3mRNA in HCC tissues, which were divided according to the cutoff of 2.51, the median value ofPBX3relative to GAPDH mRNA. Figure 5: PBX3 is a critical determinant of α2δ1 + HCC TICs. ( a , b ) The expression of PBX3 in Hep-11 and Hep-12 cells was detected at both mRNA and protein levels using qRT–PCR ( a ) and western blot ( b ), respectively. ( c , d ) The expression of PBX3 was compared between α2δ1 + and α2δ1 − fractions from indicated sources at both mRNA ( c ) and protein levels ( d ). ( e , f ) qRT–PCR ( e ) and western blot ( f ) results showing the knockdown effects of PBX3 shRNAs on the expression of PBX3 in Hep-12 cells at both mRNA and protein levels. β-actin serves as an internal control. ( g ) Sorted α2δ1 + cells from indicated sources were infected with lentiviruses harbouring PBX3 shRNAs, followed by plating 100 cells per well into 96-well plates to assay their sphere formation potential ( n =6). Data are the average±s.d. of three independent experiments. *Student’s t -test. ( h ) α2δ1 − cells from indicated sources were infected with PBX3 lentivirus and assayed for PBX3 by western blot. ( i ) FACS-sorted α2δ1 − cells from indicated sources were infected with PBX3 lentivirus and assayed for their sphere formation ability ( n =6). Data are the average±s.d. of three independent experiments. *Student’s t -test. ( j ) HE staining showing the histology of the tumours formed by α2δ1 − cells from indicated sources after PBX3 lentivirus infection. Scale bar, 100 μm. ( k ) The percentage of α2δ1-positive cells were measured using flow cytometry in PBX3 -lentivirus-infected Huh7 α2δ1 − cells compared. with vector alone control. The data are representative of three experiments. ( l ) The expression of stem cell-related genes in α2δ1 − cells overexpressing PBX3 was compared with vector alone controls using qRT–PCR. ( m ) The expression of PBX3 mRNA in HCC tissues was compared with adjacent normal tissues using qRT–PCR. *The numbers next to the horizontal lines are the median values (2 −Δ C t ) for each group. ( n , o ) Kaplan–Meier curves for the DFS and OS of patients were compared between groups with high and low levels of PBX3 mRNA in HCC tissues, which were divided according to the cutoff of 2.51, the median value of PBX3 relative to GAPDH mRNA. Full size image We then tested whether PBX3 is required for the maintenance of TIC properties by knockdown of PBX3 in α2δ1 + TICs with short-hairpin RNA (shRNA). Stable knockdown PBX3 in Hep-12 cells was achieved by infection with two lentiviruses harbouring PBX3 shRNA sequence 592 and 928, respectively, with shRNA592 having a more prominent effect on PBX3 silencing ( Fig. 5e,f ). Compared with scramble sequence, PBX3 repression led to remarkable suppression of both the spheroid formation and the tumorigenic abilities of Hep-12 cells. Moreover, similar inhibition effects on the hepatosphere formation and the tumorigenicity were obtained when α2δ1 + TICs sorted from HCC cell lines and primary tissues were infected with PBX3 shRNA lentiviruses ( Fig. 5g ; Table 2 ), demonstrating that PBX3 is necessary for the maintenance of α2δ1 + TICs’ self-renewal and tumorigenic capabilities. Table 2 The tumorigenic property of α2δ1 + and α2δ1 − HCC cells knocking down or overexpressing PBX3 . Full size table In addition, ectopic expression of PBX3 in α2δ1 − fractions sorted from HCC cell lines and primary HCC was performed to address whether PBX3 is sufficient to induce TIC-like phenotypes. Ectopic expression of PBX3 in α2δ1 − subsets ( Fig. 5h ) significantly enhanced the ability of these cells to initiate hepatosphere formation when grown in serum-free condition and to expand in subsequent serial propagations ( Fig. 5i ). Interestingly, these α2δ1 − cells overexpressing PBX3 exhibited an enhanced or newly acquired ability to initiate tumours when as few as 100 cells were injected s.c. in NOD/SCID mice compared with vector alone controls ( Table 2 ). HE staining of xenografted tumours confirmed a primary HCC phenotype ( Fig. 5j ). Importantly, primary xenografted tumours formed by these α2δ1 − cells overexpressing PBX3 could also self-renew, as demonstrated by their ability to serially transplant in secondary NOD/SCID mouse recipients ( Table 2 ). Finally, a distinct α2δ1 + subpopulation was observed following forced expression of PBX3 in α2δ1 − Huh7 cells ( Fig. 5k ). We finally address whether PBX3 could regulate the genes associated with HCC TICs. The expression of a number of HCC TIC-associated genes such as NANOG , OCT4 , ABCG2 , MDR1 and BMI1 was found to be remarkably increased following ectopic expression of PBX3 in α2δ1 − subpopulations, compared with vector controls ( Fig. 5l ). Collectively, these data demonstrate that PBX3 is sufficient to reprogramme α2δ1 − HCC cells into TICs with stem cell-like properties and is necessary for the maintenance of α2δ1 + TIC properties. Clinical significance of PBX3 in HCC patients To determine the clinical significance of PBX3 expression in HCC patients, we performed qRT–PCR analysis in 89 HCC patients. Compared with matched adjacent normal liver tissues, the expression of PBX3 mRNA was significantly upregulated in HCC tissues ( Fig. 5m ). Further analysis of 85 HCC patients with detailed follow-up data indicated that the levels of PBX3 mRNA in HCC tissues were positively correlated with the presence of hepatic cirrhosis, tumour size, rapid recurrence and short overall survival time ( Supplementary Table 3 ). Kaplan–Meier curves show that those patients with higher levels of PBX3 displayed short both disease-free and overall survival periods ( Fig. 5n,o ). Cox regression analysis identified the expression of PBX3 mRNA in HCC as an independent risk factor of poor survival for patients ( Supplementary Table 4 ). Genome-wide identification of PBX3 target genes To find the mechanisms underlying the roles of PBX3 in HCC TIC potential regulation genome widely, chromosome immunoprecipitation-sequencing (ChIP-seq) using the specific rabbit anti-PBX3 polyclonal antibody and RNA-seq were performed in SMMC7721 cell line stably overexpressing PBX3 . Model-based analysis of ChIP-Seq identified 39,508 PBX3-bound regions, which were predominantly distributed in introns, intergenic regions and promoter within 3 kb of transcription start site (TSS) for a known gene ( Fig. 6a ). Furthermore, the PBX3-binding peaks were enriched around the TSS ( Fig. 6b ). Association of PBX3-bound regions with annotated genes has identified 9,192 PBX3-bound nearest genes, reflecting an average number of 4.3 PBX3-bound regions per gene. 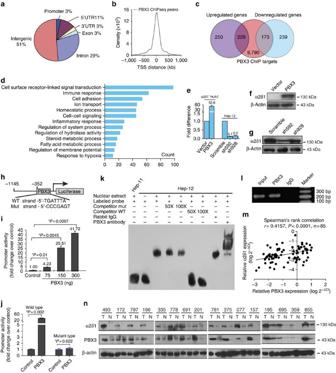Figure 6: The transcriptional programme driven by PBX3 in HCC TICs. (a) Piediagram summarizing the genomic occupancy of PBX3-bound regions as revealed by ChIP-seq. (b) Line diagram showing the distances of PBX3-bound peaks to the TSS. (c) Venn diagram illustrating direct target genes regulated by PBX3. (d) Gene Ontology (GO) term analysis of differentially regulated genes, as revealed using RNA-seq, in PBX3-overexpressed SMMC7721 cells over vector control. (e) qRT–PCR results showing α2δ1 mRNA levels inPBX3-overexpressed α2δ1−Huh7 cells andPBX3knockdown Hep-12 cells. (f,g) Western blot results demonstrating the change of endogenous α2δ1 proteins following forced expression ofPBX3in α2δ1−Huh7 cells or shRNA-mediated knockdown ofPBX3in Hep-12 cells, respectively. (h) Schematic representation of theCACNA2D1promoter that is fused to a luciferase reporter gene. The WT and mutant (Mut) sequences of the consensus potential PBX3-binding site used to makeCACNA2D1WT and Mut reporters, respectively, are indicated. (i,j) PBX3 activates the activity of the WTCACNA2D1promoter in a dose-dependent manner (i), but not that of the mutant-type promoter containing mutant consensus potential PBX3-binding site (j). Luciferase reporter assay was performed in Hep-11 cells by co-transfectionCACNA2D1reporter with either pcDNA3-PBX3or empty vector. Co-transfection of PRL-TK served as an internal control. Luciferase values were normalized to Renilla reporter activity. Data are presented as mean±s.d. of three independent experiments with triplicates. *Student’st-test. (k) EMSA analysis was performed by incubating biotin-labeled oligonucleotide target containing consensus potential PBX3-binding site with Hep-11 or Hep-12 cell lysates. (l) ChIP assay was performed with control IgG or anti-PBX3 antibody in Hep-12 cells. The precipitated DNAs were amplified with primer pairs specific for flank sequence of the PBX3-binding sites in theCACNA2D1promoter using PCR. (m) The correlation between the expression ofPBX3and its direct targetCACNA2D1in HCC tissues as detected using qRT–PCR. (n) Western blot results showing the correlation between PBX3 and α2δ1 in 16 pairs of HCC (T) and adjacent normal tissues (N). Figure 6: The transcriptional programme driven by PBX3 in HCC TICs. ( a ) Piediagram summarizing the genomic occupancy of PBX3-bound regions as revealed by ChIP-seq. ( b ) Line diagram showing the distances of PBX3-bound peaks to the TSS. ( c ) Venn diagram illustrating direct target genes regulated by PBX3. ( d ) Gene Ontology (GO) term analysis of differentially regulated genes, as revealed using RNA-seq, in PBX3-overexpressed SMMC7721 cells over vector control. ( e ) qRT–PCR results showing α2δ1 mRNA levels in PBX3 -overexpressed α2δ1 − Huh7 cells and PBX3 knockdown Hep-12 cells. ( f , g ) Western blot results demonstrating the change of endogenous α2δ1 proteins following forced expression of PBX3 in α2δ1 − Huh7 cells or shRNA-mediated knockdown of PBX3 in Hep-12 cells, respectively. ( h ) Schematic representation of the CACNA2D1 promoter that is fused to a luciferase reporter gene. The WT and mutant (Mut) sequences of the consensus potential PBX3-binding site used to make CACNA2D1 WT and Mut reporters, respectively, are indicated. ( i , j ) PBX3 activates the activity of the WT CACNA2D1 promoter in a dose-dependent manner ( i ), but not that of the mutant-type promoter containing mutant consensus potential PBX3-binding site ( j ). Luciferase reporter assay was performed in Hep-11 cells by co-transfection CACNA2D1 reporter with either pcDNA3- PBX3 or empty vector. Co-transfection of PRL-TK served as an internal control. Luciferase values were normalized to Renilla reporter activity. Data are presented as mean±s.d. of three independent experiments with triplicates. *Student’s t -test. ( k ) EMSA analysis was performed by incubating biotin-labeled oligonucleotide target containing consensus potential PBX3-binding site with Hep-11 or Hep-12 cell lysates. ( l ) ChIP assay was performed with control IgG or anti-PBX3 antibody in Hep-12 cells. The precipitated DNAs were amplified with primer pairs specific for flank sequence of the PBX3-binding sites in the CACNA2D1 promoter using PCR. ( m ) The correlation between the expression of PBX3 and its direct target CACNA2D1 in HCC tissues as detected using qRT–PCR. ( n ) Western blot results showing the correlation between PBX3 and α2δ1 in 16 pairs of HCC (T) and adjacent normal tissues (N). Full size image Compared with empty lentivirus-infected SMMC7721 cells, a total of 891 PBX3-responsive genes, including 479 upregulated (fold change >2, P <0.01) and 412 downregulated genes (fold change<0.5, P <0.01), was revealed in PBX3-overexpressed cells as detected using RNA-seq analysis ( Fig. 6c ; Supplementary Table 5 ). Database for Annotation, Visualization and Integrated Discovery (DAVID) gene ontology term analysis indicated that these genes were enriched for broad categories of biological processes ( Fig. 6d ; Supplementary Table 6 ). Notably, one of the significantly enriched gene groups was ion channels for calcium, potassium and sodium, as well as those involved in membrane potential regulation, suggesting that one of the critical mechanisms involved in PBX3-mediated TIC properties’ regulation might involve these ions’ influx/efflux. 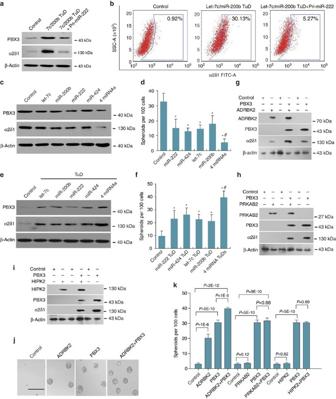Figure 7: The combinational effects of the four miRNAs and their potential targets. (a) Western blot results showing the expression of PBX3 and α2δ1 in Huh7 cells infected with indicated lentiviruses. (b) The percentage of α2δ1+cells was measured in Huh7 cells infected with indicated lentiviruses using flow cytometry. The data are representative of three experiments. (c) The expression of PBX3 and α2δ1 was assayed in α2δ1+Hep-12 cells overexpressing indicated miRNAs by western blots. (d) Hep-12 cells infected with lentiviruses harbouring indicated miRNAs were assayed for their spheroid formation ability (n=6). Data are the average±s.d. of three independent experiments. *P≤0.05 versus control; #P≤0.05 versus any other group, Student’st-test. (e) Western blot results showing the expression of PBX3 and α2δ1 in Huh7 cells following indicated miRNA knockdown. (f) The spheroid formation efficiency in Huh7 cells was measured following indicated miRNAs knockdown (n=6). Data are the average±s.d. of three independent experiments. *P≤0.05 versus control; #P≤0.05 versus any other group, Student’st-test. (g–i) Western blot results showing the expression of indicated proteins in HuH7 cells overexpressing indicated genes. β-actin serves as an internal control. (j) Representative photographs demonstrating the spheroids formed by Huh7 cells overexpressingADRBK2,PBX3 or both. Scale bar, 250 μm; (k) Huh7 cells overexpressing the indicated genes were measured for their spheroid formation efficiency. Data are the average±s.d. of three independent experiments.Pvalues were calculated by Student’st-test. Importantly, functional annotation showed that the most significantly enriched genes (243 out of the 479 upregulated genes), including SOX2 , SALL2 , NOTCH3 , WNT10A and LIN28A , were associated with embryo development ( Supplementary Table 7 ). In addition, those genes associated with HCC TICs including the TIC markers CACNA2D1 (ref. 30 ), EpCAM (ref. 38 ) and THY1 (ref. 39 ), as well as multidrug-resistant gene ABCB1 ( MDR1 ), were also among the PBX3-upregulated genes. Cross-analysis of PBX3-responsive genes with PBX3-motif-bearing PBX3-bound genes has identified 229 upregulated genes and 173 downregulated genes, representing directly activated or repressed genes by PBX3, respectively ( Fig. 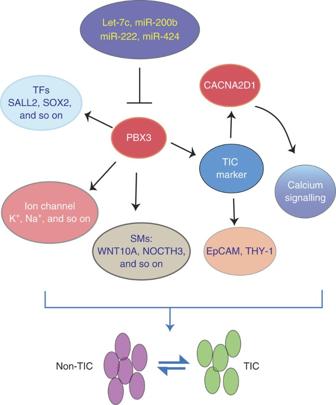Figure 8: A schematic illustration of the regulation pathway that determines the switch of HCC TICs and non-TICs. SM, signalling molecule; TF, transcriptional factor. 6c ; Supplementary Table 8 ). Many of the aforementioned genes such as CACNA2D1, EpCAM, SOX2 , SALL2 , NOTCH3 and WNT10A are among PBX3 directly activated genes, indicating that PBX3 controls an essential transcriptional programme for HCC TICs. Validation of the activation role of PBX3 on CACNA2D1 As a validation of the above RNA-seq and ChIP-seq results, we tested whether PBX3 directly activated the expression of CACNA2D1 in detail. We first detect whether PBX3 regulates the expression of endogenous α2δ1. Forced expression of PBX3 in α2δ1 − Huh7 cells resulted in the activation of α2δ1 expression at both mRNA and protein levels ( Fig. 6e,f ). On the other hand, repression of PBX3 expression in α2δ1 + Hep-12 cells led to the decrease in both α2δ1 mRNA and protein levels ( Fig. 6e,g ). We next constructed the luciferase reporter for the CACNA2D1 promoter ( Fig. 6h ) and performed luciferase reporter assay. As shown in Fig. 6i , a dose-dependent increase in the CACNA2D1 promoter-driven luciferase activity was observed in PBX3 transiently transfected Hep-11 cells over vector control. When the PBX3 potential binding consensus site in the reporter vector was mutated, the activation effect of PBX3 was no longer detected ( Fig. 6j ), indicating that the binding site of PBX3 on CACNA2D1 promoter was responsible for the activation effect of PBX3. We then carried out electrophoresis mobility shift assay using biotin-labeled probe containing the putative PBX3-binding site to test whether the potential PBX3-binding site does bind to PBX3. Incubation of the labeled WT PBX3-binding consensus oligonucleotide with the nuclear lysate of Hep-12 cells, which express high level of PBX3, clearly showed a retarded band compared with the labeled oligonucleotide without nuclear lysates or with nuclear lysates from Hep-11 cells expressing little PBX3. Furthermore, the retarded band was competed out specifically with an excess of unlabeled WT probe, and was supershifted by PBX3 antibody. In addition, the retarded band was not affected by competition with mutant PBX3-binding site oligonucleotide, or incubated with control IgG ( Fig. 6k ). We also performed ChIP assay using Hep-12 cells to verify that PBX3 actually bound to the CACNA2D1 promoter in the native state. As shown in Fig. 6l , the promoter region flanking the putative PBX3-binding motif of CACNA2D1 was successfully precipitated by PBX3 antibody as evidenced by the presence of positive PCR band in the ChIP product. As an additional supporting evidence that PBX3 activates the expression of CACNA2D1 in clinical HCC samples, the mRNA level of PBX3 was found to be positively correlated with that of CACNA2D1 in 85 HCC tissues as detected using qRT–PCR ( Fig. 6m ). Western blot results in 16 pairs of tumour and paracancerous tissues from HCC patients also demonstrate a positive correlation between the expression of PBX3 and α2δ1 at the protein level ( Fig. 6n ). MiR-222 overcomes the effects of let-7c/miR-200b knockdown Since the downregulation of let-7c and miR-200b and the upregulation of miR-222 were found extensively in HCC cells [40] , [41] , [42] , the fact that most HCC cells remain α2δ1-negative led us to propose that miR-222 could rescue the effects of let-7c/miR-200b down-regulation on the expression of PBX3 and α2δ1 in HCC cells. To test this hypothesis, we overexpressed miR-222 in Huh7 cells with let-7c and miR-200b knocked down simultaneously by respective Tud RNAs. While downregulation of let-7c and miR-200b resulted in remarkable increase in PBX3 and α2δ1 expression, further overexpression of miR-222 led to their expression decreased to the levels very close to those of parent Huh7 cells ( Fig. 7a ). Furthermore, the percentage of α2δ1 + cells increased to ∼ 30.13% following let-7c and miR-200b knockdown, while it decreased to 5.27% when miR-222 was further overexpressed ( Fig. 7b ). These results indicate that it is the combinational effect of miR-222 upregulation and let-7c/miR-200b downregulation at least that determines the expression status of α2δ1 in most HCC cells. Figure 7: The combinational effects of the four miRNAs and their potential targets. ( a ) Western blot results showing the expression of PBX3 and α2δ1 in Huh7 cells infected with indicated lentiviruses. ( b ) The percentage of α2δ1 + cells was measured in Huh7 cells infected with indicated lentiviruses using flow cytometry. The data are representative of three experiments. ( c ) The expression of PBX3 and α2δ1 was assayed in α2δ1 + Hep-12 cells overexpressing indicated miRNAs by western blots. ( d ) Hep-12 cells infected with lentiviruses harbouring indicated miRNAs were assayed for their spheroid formation ability ( n =6). Data are the average±s.d. of three independent experiments. * P ≤0.05 versus control; # P ≤0.05 versus any other group, Student’s t -test. ( e ) Western blot results showing the expression of PBX3 and α2δ1 in Huh7 cells following indicated miRNA knockdown. ( f ) The spheroid formation efficiency in Huh7 cells was measured following indicated miRNAs knockdown ( n =6). Data are the average±s.d. of three independent experiments. * P ≤0.05 versus control; # P ≤0.05 versus any other group, Student’s t -test. ( g – i ) Western blot results showing the expression of indicated proteins in HuH7 cells overexpressing indicated genes. β-actin serves as an internal control. ( j ) Representative photographs demonstrating the spheroids formed by Huh7 cells overexpressing ADRBK2 , PBX 3 or both. Scale bar, 250 μm; ( k ) Huh7 cells overexpressing the indicated genes were measured for their spheroid formation efficiency. Data are the average±s.d. of three independent experiments. P values were calculated by Student’s t -test. Full size image Synergistic effects among the four miRNAs and their targets To address whether any synergistic effects existed among the four miRNAs, we first overexpressed them simultaneously in the TIC-enriched Hep-12 cells ( Supplementary Fig. 3A–D ). The expression of PBX3 and α2δ1 ( Fig. 7c ), as well as the spheroid formation efficiency ( Fig. 7d ) were suppressed at much stronger degrees in Hep-12 cells overexpressed the four miRNAs together than the four miRNAs individually. On the other hand, the expression of PBX3 and α2δ1 ( Fig. 7e ), as well as the spheroid formation efficiency ( Fig. 7f ) increased much more significantly with the four miRNAs knocked down simultaneously in Huh7 cells, compared with individual knockdown of them ( Supplementary Fig. 3E–H ). These data indicate that synergistic effects do exist among the four miRNAs. We then tested whether other common targets of the four miRNAs play any roles in TIC potential regulation, and whether there is any synergistic effect among them. We have selected three potential target genes, ADRBK2 (also known as GRK3 ), PRKAB2 and HIPK2 , which have been reportedly related to cancer [43] , [44] , [45] , for further study. Of the three genes, only ADRBK2 was found to be able to induce Huh7 cells to acquire in vitro self-renewal ability as evidenced by increased spheroid formation efficiency, as well as to activate the expression of α2δ1, although at a lesser degree compared with PBX3 . Furthermore, ADRBK2 could act synergistically with PBX3 , reprogramming Huh7 cells to acquire enhanced spheroid formation ability and elevated α2δ1 expression ( Fig. 7h–k ). The data indicate that at least two of the four miRNAs’ common targets can work synergistically to determine the HCC TIC potential. Taken together, all these results demonstrate that the downregulation of a set of miRNAs (let-7c, miR-200b, miR-222 and miR-424) has led to one of their direct targets, PBX3 , maintained above certain threshold, which in turn transcriptionally activates the expression of genes critical for stemness determination to maintain the HCC TIC phenotypes ( Fig. 8 ). Figure 8: A schematic illustration of the regulation pathway that determines the switch of HCC TICs and non-TICs. SM, signalling molecule; TF, transcriptional factor. Full size image Functional screening genome widely of miRNAs involved in the regulation of TICs was hindered by limited number of TICs available from a given tumour, and by their unstable characteristics in regular culture condition. The fact that most of the recurrent HCC-originated Hep-12 cells remain as TICs even with prolonged in vitro culture has led to the identification of a TIC population expressing the α2δ1 subunit [29] , [30] . Here we developed a protocol by combining genome-wide miRNA profiling with soft-agar functional screening assay based on the Hep-12 cell line, to identify miRNAs that suppress the HCC TIC fate and have successfully identified a set of miRNAs, including four most effective miRNAs (let-7c, miR-200b, miR-222 and miR-424) that suppress the stemness and tumorigenicity of α2δ1 + HCC TICs. This represents an efficiently functional screening strategy to identify all the possible miRNAs that control the properties of HCC TICs, and can be easily adopted to screen the key molecules involved in the regulation of HCC TIC properties. Of the four most effective miRNAs identified, let-7c and miR-200b belong to the let-7 and miRNA-200s families, respectively, of which the tumour-suppressor roles in TICs have been well appreciated [8] , [23] , [46] , while miR-222 and miR-424 were first identified as TIC-suppressing miRNAs despite a tumour-suppressor role of both miRNAs has been identified in a number of cancers other than HCC [47] , [48] , [49] , [50] . Paradoxically, miR-222 was previously regarded as oncogene in some reports because it could enhance some tumour cell growth by targeting CDK inhibitor p27 in vitro , and was found to be upregulated in HCC and some other types of cancers [42] , [51] , [52] ; however, its tumour-promoting role was rarely validated in vivo . Our data support miR-222 to be a tumour suppressor in HCC by controlling the stemness and tumorigenicity of α2δ1 + TICs, further confirming that the roles of miRNAs are cell context-dependent [50] . The study also indicates that a tumour suppressor on TICs was not necessarily downregulated in tumour tissues because the level reflects the status of the abundant non-TICs. Most of the previous studies on miRNAs focused on single miRNA that targets one or more genes. Here we demonstrated that four downregulated miRNAs could target PBX3 directly and synergistically at the transcriptional level to control the stemness and tumorigenicity of α2δ1 + HCC TICs. Although knockdown of any of the four miRNAs could induce a TIC phenotype of α2δ1 − cells, the facts that each of the four miRNAs alone is enough to suppress the TIC properties, and that those cells expressing decreased levels of let-7c and miR-200b, and elevated level of miR-222 remain to be non-TICs suggest that all of the miRNAs negatively regulate PBX3 need to be downregulated to activate α2δ1 + TICs. Furthermore, the four miRNAs could potentially regulate more common targets other than PBX3 ; it is interesting to determine whether all these targets also contribute to the TIC potential determination, and if so, whether they work synergistically or antagonistically with PBX3. So far, ADRBK2, another common target of the four miRNAs, was found to work synergistically with PBX3 at least. Nevertheless, our current results indicate that the combination of multiple miRNAs that target the same gene should be considered when miRNAs involved in certain biological processes are investigated [53] . PBX3 has been observed to be aberrantly overexpressed in a variety of tumours [54] , [55] , [56] , [57] , [58] ; however, little is known about its biological roles in tumorigenesis and progression. Our current study demonstrates that PBX3 plays determinant roles in HCC TIC properties, in particularly, controlling directly the expression of TIC surface markers α2δ1 and EpCAM , stem cell master genes SOX2 and SALL2 , as well as regulating the self-renewal and tumorigenicity potential. This observation is in consistent with the previous notion that the TALE homeodomain protein MEIS1 served a major role in establishing leukaemia stem cell potential and in determining leukaemia stem cell frequency probably by forming a complex with PBX proteins [59] . It would be interesting to further determine whether the roles of PBX3 in determining the TIC potential is also dependent on the interaction with other TALE homeodomain proteins such as MEIS and HOX family members. In summary, we have identified four miRNAs that serve as negative regulators of α2δ1 + HCC TICs by targeting directly PBX3 , which drives a stem cell-like transcriptional programme, including activation the genes related to calcium signalling, to enable HCC cells to reprogramme into TICs. Restoration of any of these miRNAs or interfering the expression/blocking the function of PBX3 in HCC cells may represent an promising strategy for future HCC treatment by reducing TICs. Future work is needed to address the driving events in the α2δ1 + cell-induced HCC, especially how the four miRNAs are deregulated in the α2δ1 + HCC TICs. Cell lines and clinical samples HCC cell lines Hep-11 and Hep-12 were established by primary culture of a patient’s primary and recurrent liver cancer tissues, respectively [29] . The Huh7, HepG2 and SMMC7721 cell lines were originated from Japan Society for the Promotion of Science (Tokyo, Japan), American Type Culture Collection (Manassas, VA) and the Second Military Medical University of China (Shanghai, China), respectively. All cell lines were cultivated in RPMI 1640 medium supplemented with 10% fetal bovine serum, 100 U ml −1 penicillin and 100 mg ml −1 streptomycin (Invitrogen, Grand Island, NY, USA) in a humidified atmosphere of 5% CO 2 at 37 °C. They were authenticated using polymorphic short tandem repeat loci and were tested for no mycoplasma contamination before the study initiated. Primary HCC specimens and matched adjacent normal tissues were collected and snap-frozen into liquid nitrogen from patients at the time of hepatectomy performed at the Beijing Cancer Hospital with written informed consent. Some primary HCC tissues were minced and dissociated into single cells by collagenase IV digestion for TIC isolation, or xenografted into NOD/SCID mice for repeated use. Acquisition and use of these tissues were approved by the Ethics Committee of Peking University Cancer Hospital. Immunofluorescent staining and flow cytometry analysis Cells were detached from culture by 0.02% EDTA/PBS or were dissociated from primary or xenografted tumours by mechanical homogenization, and were stained by rabbit anti-α2δ1 polyclonal antibody (1:100 dilution, Sigma-Aldrich, St Louis, MO, # HPA008213), or Mab1B50-1 (ref. 30 ; 40 μg μl −1 ), which were pre-labeled using the Lightning- Link PE-Cy5 Labeling Kit (Innova Biosciences Ltd, Cambridge, UK) at 4 °C for 30 min. Labeled samples were analysed or sorted on a FACSAria II flow cytometer (BD Biosciences, San Jose, CA). Quantitative μParaflo miRNA microarray analysis miRNA microarray assay was carried out using a service provider (LC Sciences, Houston, TX). The assay started from 5 μg total RNA sample, which was size-fractionated using a YM-100 Microcon centrifugal filter (Millipore, Billerica, MA), and the small RNAs (<300 nucleotides) isolated were 3′-extended with a poly(A) tail using poly(A) polymerase (NEB, Beverly, MA). An oligonucleotide tag was then ligated to the poly(A) tail for carrying out fluorescent dye staining later. Two different tags were used for the two RNA samples in dual-sample experiments. Hybridization was conducted overnight on a μParaflo microfluidic chip (miRHuman_13.0) using a microcirculation pump (Atactic Technologies, Houston, TX). On the microfluidic chip, each detection probe consisted of a chemically modified nucleotide-coding segment complementary to target miRNA (from miRNABase, http://microrna.sanger.ac.uk/sequences/ ) or other RNA (control sequences). Hybridization used 100 μl 6 × SSPE buffer (0.90 M NaCl, 60 mmol l −1 Na 2 HPO 4 , 6 mmol l −1 EDTA, pH 6.8) containing 25% formamide at 34 °C. After RNA hybridization, tag-conjugating Cy3 and Cy5 dyes were circulated through the microfluidic chip for dye staining. Fluorescence images were collected using a laser scanner (GenePix 4000B, Molecular Devices, Sunnyvale, CA) and digitized using Array-Pro image analysis software (Media Cybernetics, Rockville, MD). Spheroid formation assay Spheroid formation was performed by plating 100 cells per well into 96-well ultra-low attachment plate (Corning Incorporated Life Sciences, Acton, MA) in serum-free DMEM/F12 medium (Invitrogen), supplemented with B27 (1:50; Invitrogen), 20 ng ml −1 bFGF, 10 ng ml −1 HGF (Peprotech, Rocky Hill, NJ) and 1% methylcellulose (Sigma-Aldrich). Cells were incubated in a CO 2 incubator for 2–3 weeks and spheres were counted under a stereomicroscope (Olympus, Shinjuku-ku, Tokyo, Japan). Tumorigenicity assay For the assessment of tumour-formation abilities, cells were suspended in 50 μl of plain RPMI1640 and Matrigel (BD Biosciences) mix (1:1) and transplanted s.c. into the armpit of 4- to 6-week-old NOD/SCID male and female mice (NOD.CB17- prkdc scid /NcrCrl, Vitalriver, Beijing, China). Tumour formation was monitored weekly. All the animal protocols were performed under a Peking University Cancer Hospital Animal Care and Use Committee-approved protocol. Total RNA extraction and qRT–PCR Total RNAs were isolated with the miRNeasy Mini kit (Qiagen, Valencia, CA). For mature miRNA quantification, 50 ng total RNA was polyadenylated by polyA polymerase (NEB), followed by reverse transcription with an oligo-dT adapter primer. For mRNA detection, cDNA was synthesized from total RNA using oligo(dT) 15 primers and Moloney murine leukaemia virus reverse transcriptase (Invitrogen, Carlsbad, CA). Real-time PCR was performed using SYBR Green PCR Master Mix (Toyobo, Osaka, Japan) on an ABI7500 PCR machine. Results were normalized to U6 for miRNA detection and GAPDH for mRNA measurement. Fold change was calculated by the 2 −ΔΔ C t method where Δ C t = C t(Target) − C t(Reference) . All the primers were listed in Supplementary Table 9 . The specificity of the PCR was confirmed by melting curves and PCR product sequencing. Soft-agar assay Approximately 1,000 cells of each miRNA-transfected cell pool were plated in 0.5 ml of 0.3% (w/v) Noble Agar (Difco, Detroit, MI) in culture medium on a solidified basal layer agar (0.5 ml of 0.5% agar in medium) per well in 24-well culture plates, 6 wells per group. At 2 weeks after seeding, the colonies that contain at least 50 cells were counted under a microscope. Fluorescence in situ hybridization of miRNAs In situ hybridization of miRNAs was performed according to the miRCURY LNA microRNA ISH Protocol by using specific miRNA probes labeled with Digoxin (Exiqon, Vedbaek, Denmark). Images were captured on a Leica SP5 confocal microscope (Leica, Wetzlar, Germany). Vector construction All the constructs were made by standard DNA recombination techniques. The human pri-miRNA sequences containing each pre-miRNA and flanking sequence on both sides of pre-miRNA were amplified using PCR from genomic DNA using primers listed in Supplementary Table 9 , and were subsequently cloned into pcDNA3.0, and/or lentiviral shuttle vector plenti6 (Invitrogen), or tetracycline-regulated plenti6-TREpitt vector, which was constructed in our previous study. The construction of PBX3 expression vector was described in our earlier paper [36] . For knockdown of miRNA expression, TuD RNAs against let-7c (5′-GGATCCgacggcgctaggatcatcaacaaccatacaaccatcttactacctcacaagtattctggtcacagaatacaacaaccatacaaccatcttactacctcacaagatgatcctagcgccgtcttttttCTCGAG-3′), miR-200b (5′-GGATCCgacggcgctaggatcatcaactcatcattaccaatctggcagtattacaagtattctggtcacagaatacaactcatcattaccaatctggcagtattacaagatgatcctagcgccgtcttttttCTCGAG-3′), miR-222 (5′-GGATCCgacggcg ctaggatcatcaacacccagtagccatctagatgtagctcaagtattctggtcacagaatacaacacccagtagccatctagatgtagctcaagatgatcctagcgccgtcttttttCTCGAG-3′) and miR-424 (5′-GGATCCgacggcgctag gatcatcaacttcaaaacatgaatctattgctgctgcaagtattctggtcacagaatacaacttcaaaacatgaatctattgctgctgcaagatgatcctagcgccgtcttttttCTCGAG-3′) were designed according to ref. 32 . For PBX3 knockdown constructs, two shRNA sequences, including shRNA592 (5′-GAGATTGAAAGAATGGTGGGC-3′) and shRNA928 (5′-AGACGGCCGTGACAGCTGCAC-3′), were designed. These TuD RNAs and shRNAs were cloned into lentiviral shuttle vector plenti6-U6. For miRNA sensor vectors, the 3′UTRs of PBX3 containing WT or mutant mature miRNA complementary sequences were cloned into the luciferase reporter vector. For CACNA2D1 reporter vector, the putative promoter region containing potential PBX3-binding site was amplified using PCR and cloned into PGL3-basic vector (Promega Corporation, Madision, WI) fused to a luciferase reporter gene. For construction of the PBX3-binding site mutant CACNA2D1 promoter-driven reporter, site-directed mutagenesis was carried out to obtain the mutant sequence of the promoter, and was then subcloned into the same vector. The PCR primers used for making these constructs are listed in Supplementary Table 9 . All the constructs were confirmed by sequencing. Transfection of pcDNA3.0 constructs into Hep-12 cells was performed using Lipofectamine 2000 reagent (Invitrogen) and then stable cell lines were obtained by selection with 500 μg ml −1 G418 (Invitrogen). Lentiviral constructs were transfected with the ViraPower Packaging Mix (Invitrogen) into 293FT cells to generate lentivirus. Cells infected with virus are selected by 5 μg ml −1 blasticidin (Invitrogen) and/or 500 μg ml −1 G418. The pool of antibiotic-resistant cells were used for subsequent assay. Western blot analysis Cells were lysed in radioimmunoprecipitation assay buffer (Suolaibo Biotechnology Co. Ltd, Shanghai, China) containing complete protease and phosphatase inhibitor cocktail (Roche, Mannheim, Germany). Cell lysates were then resolved through 10% SDS–PAGE, transferred on polyvinylidene difluoride membrane (Millipore) and probed by rabbit anti-PBX3 (1:3,000 dilution, Abcam, Cambridge, UK, # Ab109173), mouse anti-α2δ1 (1:3,000 dilution, Sigma-Aldrich, # HPA008213) or mouse anti-β-actin (1:50,000 dilution, Roche, # 1378996), followed by incubation with horseradish peroxidase (HRP)-conjugated goat anti-rabbit(1:100,000 dilution, Jackson ImmunoResearch Laboratories, West Grove, PA, # 111-035-003) or anti-mouse IgG (1:100,000 dilution, Jackson ImmunoResearch Laboratories, # 115-035-003) secondary antibody. Signals were detected with Immobilon Western Chemiluminescent HRP substrate (Millipore). Images have been cropped for presentation. Full-size images are presented in Supplementary Figs 4–7 . Luciferase reporter assay To determine relative luciferase activity, cells were seeded into 24-well plates. Each reporter construct was co-transfected with pRL-TK plasmid expressing renilla luciferase, and pri-miRNA or PBX3 expression vector using lipofectamine 2000 (Invitrogen). After 24 h, cell lysates were made using 1 × passive lysis buffer (Promega Corporation) according to the manufacturer’s instructions. Firefly and Renilla luciferase activities in cell lysates were measured by a FLUOstar Optima illuminometer (BMG Labtech, Offenburg, Germany) using the dual-luciferase reporter assay kit (Promega). Firefly luciferase activity was normalized to that of renilla luciferase for each sample. Chromatin immunoprecipitation assay The chromatin immunoprecipitation (ChIP) assay was performed with the ExactaChIP Kit according to the manufacturer's instruction (R&D Systems, Minneapolis, MN). Briefly, Hep-12 cells or PBX3-transfected Huh7 cells were formaldehyde-crosslinked, and the DNA was sheared by sonication. The crosslinked whole-cell extract was used for immunoprecipitation with PBX3 antibody or control IgG. After overnight immunoprecipitation, each sample was washed with washing buffers. The DNA was eluted and purified using the PCR Purification Kit from Qiagen. PCR was performed with primers specific for human CACNA2D1 (forward: 5′-TTGCCTAAGAAGCCAGACGG-3′, reverse: 5′-AGGGCGACTTTGGAAACAGAC-3′). The ChIP products were sequenced using Illumina Hi-Seq 2000 (Illumina Inc., San Diego, CA) by a service provider (BIOPICS, Peking University, Beijing, China). ChIP-seq data analysis For ChIP-seq analysis, Illumina sequencing short reads were aligned against the Human Reference Genome (assembly hg19) using the Burrows–Wheeler Aligner [60] tool with default settings. Only unique non-duplicate reads were retained. Peaks, areas where there were significantly more enriched reads mapped in the ChIP sample than the input, were determined using MACS [61] with the parameters of P value 0.00001 and false discovery rate 5%. The Bedtools software [62] was used to determine the genes closest to PBX3-binding peaks and to calculate the distance between these peaks from TSS of their closest genes. Electrophoretic mobility shift assay Electrophoretic mobility shift assay (EMSA) was performed using the LightShift chemilluminescent EMSA kit (Pierce, Rockford, IL) essentially the same as described [63] . The double-stranded oligonucleotide used as a probe for EMSA corresponds to the following sequence in the putative PBX3 WT binding site of the CACNA2D1 promoter region, 5′-TCCTCCC TGATTTAT TCCCCCG-3′. The consensus sequence TGATTTA was changed to TCGAGCG in the respective mutant PBX3-binding motif used in the competition experiments. Probes were end-labeled with biotin. Reaction mixture of 20 μl containing binding buffer, 5% glycerol (v/v), 5 mM MgCl 2 , 50 ng μl −1 Poly(dI·dC), 0.05% NP-40, 150 mM KCl, 20 fmol probe and 10 μg nuclear extract, which was prepared using NE-PER Nuclear and Cytoplasmic Extraction (Pierce, Philadelphia, PA), were incubated at room temperature for 30 min. For competition assays, excess unlabeled double-strand nucleotides were added to the reaction mixture. Either control IgG or PBX3 polyclonal antibody was included in the reaction mixture for super-shift assay. The DNA–protein complexes were separated on 6% native polyacrylamide gel in 0.5 × TBE and were electrophoretically transferred on positively charged nylon membrane. DNA and membrane were crosslinked at 120 mJ cm −2 using ultraviolet crosslinker at 254 nm. Signals were detected using the Chemiluminiscent Nucleic Acid Detection module (Pierce) according to the manufacturer's protocol. RNA-seq data analysis Total RNA was isolated from SMMC7721 cells infected with PBX3 expression and control vector lentiviruses. Samples were sequenced on an Illumina Hi-Seq 2000 with 100-bp paired end. FASTQ sequence reads were aligned to the human reference genome (hg19) with the Burrows–Wheeler AlignerBWA tool at default settings [60] . The expression level of each gene was expressed as number of reads per kilobase per million mapped reads calculated according to the formula published in ref. 64 . Exact test based on a Poisson model was used for differential expression gene analysis. The fold change of the expression level of each gene was calculated as the ratio of PBX3 overexpression to vector alone control. Genes with P <0.01, fold change >2 were considered to be upregulated genes by PBX3. Genes with P <0.01, fold change value <0.5 were considered to be downregulated genes by PBX3. Gene ontology analysis of PBX3 target genes was performed using the NIH DAVID ( http://david.abcc.ncifcrf.gov/ ). Statistical analysis All data were analysed with methods defined in the text using SPSS 13.0. A P value ≤0.05 was considered statistically significant. Accession codes. The miRNA microarray and PBX3 transcriptome (ChIP-seq and RNA-seq) data sets have been deposited in the Gene Expression Omnibus database with the accession IDs GSE71004 and GSE71262 , respectively. How to cite this article: Han, H. et al . PBX3 is targeted by multiple miRNAs and is essential for liver tumour-initiating cells. Nat. Commun . 6:8271 doi: 10.1038/ncomms9271 (2015).